Full open-framework batteries for stationary energy storage New types of energy storage are needed in conjunction with the deployment of renewable energy sources and their integration with the electrical grid. We have recently introduced a family of cathodes involving the reversible insertion of cations into materials with the Prussian Blue open-framework crystal structure. Here we report a newly developed manganese hexacyanomanganate open-framework anode that has the same crystal structure. By combining it with the previously reported copper hexacyanoferrate cathode we demonstrate a safe, fast, inexpensive, long-cycle life aqueous electrolyte battery, which involves the insertion of sodium ions. This high rate, high efficiency cell shows a 96.7% round trip energy efficiency when cycled at a 5C rate and an 84.2% energy efficiency at a 50C rate. There is no measurable capacity loss after 1,000 deep-discharge cycles. Bulk quantities of the electrode materials can be produced by a room temperature chemical synthesis from earth-abundant precursors. New renewable energy sources such as solar and wind power are fundamentally different from conventional energy generation from fossil fuels because of their inherent intermittency [1] . The power output of solar and wind farms is limited both by diurnal cycles and short-term seconds-to-minutes volatility due to rapid changes in cloud cover and wind conditions [2] . The scientific community, industry advocates, and policy makers have repeatedly called for fast-acting energy storage in support of volatile renewable energy sources [1] , [2] , [3] , [4] . Energy storage is needed both for diurnal load balancing and the smoothing of intermittent spikes or drops in power production [5] . Energy storage systems used for this application must be deployable across the grid, have extraordinarily long cycle life, be capable of high power charge and discharge in minutes, have very high energy efficiency and, above all, have low capital and lifetime costs. A new kind of energy storage technology is needed for short-term grid storage applications, as existing technology struggles to meet the needs of these applications at a reasonable price [1] , [3] , [4] , [5] . Pumped hydroelectric power is the current industry standard for grid energy storage, but new facilities are location dependent and have very high capital costs. Both mechanical flywheels and ultracapacitors provide the long cycle life, high power, and high energy efficiency needed to smooth volatile renewable energy sources. However, their extraordinarily high costs on a Watt-hour basis have limited their use on the grid thus far. Two battery technologies that are promising for low-rate grid storage applications are sodium sulphur (NaS) and flow batteries. Unfortunately, neither of these types of batteries can operate at high rates, precluding their use for transient applications. Of the existing energy storage technologies, lead acid and lithium-ion batteries are more attractive for transient grid applications, such as short-term smoothing of solar and wind, and both of these technologies have demonstrated some success in grid-scale applications [5] . Barnhart et al . [6] , [7] recently introduced a new metric to evaluate the energetic performance of different storage technologies on the grid. According to their analysis, the two primary factors that are preventing present forms of electrochemical energy storage from being used extensively on the grid are their limited cycle life and high embodied energy (that is, the energy required to build a unit of stored energy). The reason is that previous technologies were never specifically designed to meet the demands of the grid but were instead adapted from other applications in which volumetric/specific energy and power are the key requirements. We recently demonstrated promising results with a new family of battery electrode materials based on the common, inexpensive Prussian Blue pigment [8] , [9] , [10] , [11] . Electrodeposited thin films of these materials have received substantial study in the past for their electrochromic properties, beginning with the pioneering work of Neff [12] , [13] . Prussian Blue analogues have also been studied for use as battery electrodes, most commonly as thin films in aqueous electrolytes, but also as cathodes in organic electrolyte lithium-ion cells [12] , [14] , [15] , [16] , [17] , [18] , [19] , [20] , [21] , [22] , [23] , [24] . The open-framework (OF) structure of Prussian Blue analogues is fundamentally different from other insertion electrode materials because of its large channels and interstices. This structure is composed of a face-centred cubic framework of transition metal cations where each cation is octahedrally coordinated to hexacyanometallate groups ( Fig. 1 ) [25] , [26] , [27] . For instance, in the copper hexacyanoferrate cathode, sixfold carbon-coordinated iron and sixfold nitrogen-coordinated copper are linked by CN ligands. Large interstitial ‘A sites’ within the structure can accommodate zeolitic water and hydrated alkali ions. This results in a general chemical formula of A x PR(CN) 6 ·nH 2 O, where A is an alkali cation such as K + or Na + , P is a transition metal cation such as Cu 2+ , Ni 2+ or Fe 3+ and R(CN) 6 is a hexacyanometallate anion such as Fe(CN) 6 3− , Mn(CN) 6 3− or Cr(CN) 6 3− . Both the P-site transition metal cation and the R(CN) 6 3− hexacyanometallate anion can be electrochemically active in this structure, hence, in this work, we adopt a notation of the general form P I/J —N≡C—R K/L , where I, J, K and L are valence states of the P and R cations. 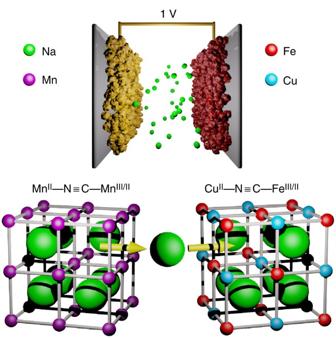Figure 1: Symmetric open-framework cell schematic. This new type of safe, fast, inexpensive, long-cycle life aqueous electrolyte battery relies on the insertion of sodium ions into the copper hexacyanoferrate (CuII—N≡C—FeIII/II) cathode and a newly developed manganese hexacyanomanganate (MnII—N≡C—MnIII/II) anode, each of which have the same open framework crystal structure. Figure 1: Symmetric open-framework cell schematic. This new type of safe, fast, inexpensive, long-cycle life aqueous electrolyte battery relies on the insertion of sodium ions into the copper hexacyanoferrate (Cu II —N≡C—Fe III/II ) cathode and a newly developed manganese hexacyanomanganate (Mn II —N≡C—Mn III/II ) anode, each of which have the same open framework crystal structure. Full size image The Prussian Blue framework structure has wide channels between the A sites, allowing rapid insertion and removal of Na + , K + and other ions from aqueous solutions. In addition, there is little lattice strain during cycling because the A sites are larger than the hydrated ions that are inserted and removed from them. The result is an extremely stable electrode: over 40,000 deep discharge cycles were demonstrated in the case of the Cu II —N≡C—Fe III/II cathode [10] . We later showed that related cathode materials including nickel hexacyanoferrate (Ni II —N≡C—Fe III/II ) [11] also have a very long cycle life when operated in a wide variety of aqueous alkali-ion electrolytes [8] , and that their reaction potentials can be controlled by altering their composition [9] . These OF structure cathodes are ideally paired with an anode that has comparable cycle life and kinetics to avoid a substantial constraint in the performance of the full battery. The activated charcoal used in commercial ultracapacitors has these properties, and we recently showed that it could be successfully combined with the Cu II —N≡C—Fe III/II cathode in an asymmetric cell [28] . However, the low specific and volumetric capacity of capacitive electrodes such as activated charcoal severely limited the specific energy and energy density of this cell. These limitations motivated us to look for anode materials with the same OF crystal structure (and the pertaining attractive properties), but with an insertion potential close to the standard hydrogen electrode (SHE). In this work, we demonstrate a new symmetric battery that uses OF materials for both its cathode and anode ( Fig. 1 ). In a few prior instances, devices of this type have been studied [22] , [23] . However, in most cases those batteries used impractically small electrodeposited thin film electrodes and used Prussian Blue itself as the anode (resulting in a very low cell voltage of about 0.6 V). They also had poor mass-balancing that resulted in the overcharge of one electrode and rapid capacity loss [22] , [23] . In contrast, in this work we demonstrate the use of manganese hexacyanomanganate (Mn II —N≡C—Mn III/II ) as an anode material that has a low reaction potential, around 0 V vs SHE, and when combined with cathodes such as Cu II —N≡C—Fe III/II , yields a useful full cell voltage of about 1 V. The electrodes in this battery can be synthesized in bulk and when operated in an appropriate aqueous electrolyte show extremely long cycle life, fast kinetics, and high efficiency, resulting in a full battery cell that can be an attractive candidate for use in large scale energy storage. Copper hexacyanoferrate cathode In our previous studies we demonstrated that copper hexacyanoferrate Cu II —N≡C—Fe III/II electrodes are promising for grid-scale energy storage applications because of their ultralong cycle life (83% capacity retention after 40,000 cycles), high power (67% discharge capacity available at 80C), high energy efficiency and potentially very low cost [7] . Copper hexacyanoferrate reacts with Na + by a single-phase insertion reaction: The standard potential of this reaction is 0.85 V with respect to the standard hydrogen electrode (SHE), which makes it an ideal material to use as a cathode in aqueous electrolytes. The material used in the experiments described here was synthesized in its oxidized form (Cu II —N≡C—Fe III , brown) with the room temperature co-precipitation method previously described and reported in the methods section. X-ray diffraction (XRD), scanning electron microscopy (SEM) and transmission electron microscopy (TEM) results are shown in Fig. 2d–f and discussed below for the sake of comparison with the Mn II —N≡C—Mn III anode. The composition of the as-synthesized material was determined by elemental analysis and ion coupled plasma mass spectrometry (ICP-MS) to be K 0.05 Cu[Fe(CN) 6 ] 0.67 · 0 .33 ·2.83H 2 O ( =Fe(CN) 6 vacancy). The as-synthesized CuHCF has a fractional initial charge state because fully oxidized CuHCF has a potential high enough that it can be reduced by water. A reductive titration method was developed to controllably reduce CuHCF to a desired oxidation state and open circuit potential using Na 2 S 2 O 3 , in the presence of an excess of potassium ions [28] . The fully reduced CuHCF (dark purple) had a composition of Na 0.036 K 0.40 Cu[Fe(CN) 6 ] 0.60 · 0.4 ·3.17 H 2 O. The X-ray photoelectron spectroscopy (XPS) spectra of both oxidized and reduced powders are reported in the Supplementary Information ( Supplementary Fig. S2 ). 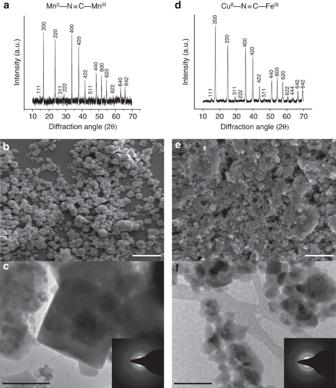Figure 2: Manganese hexacyanomanganate and copper hexacyanoferrate physical characterization. X-ray diffraction patterns of (a) MnII—N≡C—MnIIIand (d) CuII—N≡C—FeIII. Bulk synthesis of CuII—N≡C—FeIIIand MnII—N≡C—MnIIIat room temperature by co-precipitation results in a highly crystalline material. SEM shows particles of the order of 500 nm for the MnII—N≡C—MnIII(b, scale bar=5 μm) and 20–50 nm for the CuII—N≡C—FeIII(e, scale bar, 1 μm). These results are consistent with those of TEM of the MnII—N≡C—MnIII(c, scale bar. 500 nm) which show crystalline, faceted nanoparticles and CuII—N≡C—FeIII(f, scale bar, 100 nm). Figure 2: Manganese hexacyanomanganate and copper hexacyanoferrate physical characterization. X-ray diffraction patterns of ( a ) Mn II —N≡C—Mn III and ( d ) Cu II —N≡C—Fe III . Bulk synthesis of Cu II —N≡C—Fe III and Mn II —N≡C—Mn III at room temperature by co-precipitation results in a highly crystalline material. SEM shows particles of the order of 500 nm for the Mn II —N≡C—Mn III ( b , scale bar=5 μm) and 20–50 nm for the Cu II —N≡C—Fe III ( e , scale bar, 1 μm). These results are consistent with those of TEM of the Mn II —N≡C—Mn III ( c , scale bar. 500 nm) which show crystalline, faceted nanoparticles and Cu II —N≡C—Fe III ( f , scale bar, 100 nm). Full size image Electrolyte considerations Prussian Blue analogues are known to be more stable at acidic pH than in neutral and basic pH, as ligand exchange between the CN − ligands and OH − ions results in the dissolution and destruction of the Prussian Blue structure [29] . This trace solubility is the dominant loss mechanism during their operation in both battery electrodes and electrochromic devices, thereby acidic pH has been found to extend the lifetimes of these devices [30] . However, the reductive electrolysis of water to H 2 occurs at higher potentials in acid, which in turn limits the use of anodes with low reaction potentials. Moreover, acidic conditions are undesirable for practical reasons, including current collector corrosion, cell packaging and safety. Neutral 10 M NaClO 4 was adopted as the electrolyte of choice for this study because the neutral pH results in a low potential for H 2 evolution, and the high salt concentration of this electrolyte also limits the trace solubility of Prussian Blue analogues. The neutral pH of this solution results in a relatively low equilibrium potential of 0.787 V for O 2 evolution with respect to the standard hydrogen electrode (SHE). Although this is lower than the reaction potential of the Cu II —N≡C—Fe III/II cathode, in practice, O 2 evolution does not occur at an appreciable rate below 1.2 V vs SHE in this electrolyte thanks to the combination of perchlorate anion adsorption, a decrease in the chemical activity of water, and increased viscosity of the solution. Galvanostatic cycling data and cycle life for the Cu II —N≡C—Fe III/II cathode using an activated carbon counter electrode are reported in the Supplementary Information ( Supplementary Fig. S4 ). Finally, the choice of an aqueous, neutral electrolyte results in a safe battery, with no flammability or explosion hazards and limited corrosion. Open-framework anodes The development of a suitable anode has proven to be challenging for a wide variety of aqueous electrolyte batteries, for several reasons [31] . Very few of the transition metal oxides and phosphates typically used to intercalate Li + and Na + have reaction potentials between –0.5 V and 0 V vs SHE, the optimal range for anodes in aqueous electrolytes [32] . Some, such as VO 2 and LiV 3 O 8 , are partially soluble [33] . If the anode potential is slightly too low, as in the case of the NASICON A 1+x Ti 2 (PO 4 ) 3 (A=Li, Na), then the low coulombic efficiency of the anode will result in overcharge of the cathode, unless the cathode potential is tuned to result in commensurate O 2 evolution [34] . Other intercalation electrodes such as transition metal sulphides are potentially subject to irreversible hydrolysis. A major advantage of an aqueous electrolyte system is its low cost. This precludes the use of tungsten and molybdenum oxide bronzes and indium oxide that have all been used in aqueous electrolyte electrochromic devices [35] . Development of metal-hydride anodes with high enough reaction potentials for use in neutral pH may be possible, but the lanthanides they typically contain are generally too expensive. The use of a Prussian Blue analogue as an anode in aqueous alkali ion batteries could overcome these challenges: several materials in this family have reaction potentials in the desired range, and they can be produced rapidly in bulk from inexpensive precursors. To maximize the voltage and, therefore, the stored energy of an aqueous battery, the reaction potentials of the anode and cathode must be as close as possible to the potentials for H 2 and O 2 evolution in the chosen electrolyte. In their early work, Dostal and Scholz [36] investigated many Prussian Blue analogues in aqueous electrolytes. Table 1 summarizes the Prussian Blue analogues that have a potential close to the lower stability limit of pH-neutral aqueous electrolytes. Table 1 Standard reduction potential of feasible hexacyanometallate anodes in a 1M K + electrolyte [36] , [47] . Full size table The energy stored in a battery scales with the voltage, hence lower anode reaction potentials are desirable. However, the equilibrium H 2 reduction potential in neutral pH is −0.413 V, hence anodes that operate at potentials appreciably lower than this suffer from poor coulombic efficiency and cannot be used. Cr II —N≡C—Mn III/II would result in an impractically low battery voltage of 0.6 V if paired with the Cu II -N≡C-Fe III/II cathode. Fe II —N≡C—Mn III/II cannot be used in aqueous electrolytes because of rapid Fe—N/Mn—C isomerization that results in the formation of the Mn II -N≡C-Fe III/II cathode [37] , [38] . Of the anodes synthesized in this study, Cr II —N≡C—Mn II/I is the most attractive for use in an aqueous battery at neutral pH, as its lower reaction occurs at −0.312 V vs SHE ( Fig. 3a ). Unfortunately, synthesis of phase-pure Cr II —N≡C—Mn III is challenging due to the tendency of the Cr 2+ to hydrolyze and Mn 3+ to disproportionate. For this reason, the crystallinity of Cr II —N≡C—Mn III was too poor to allow a reliable calculation of its lattice parameter, and, although its electrochemical activity was successfully measured ( Fig. 3a ), its specific capacity was less than half of the 60 mAh g −1 typically observed for Prussian Blue analogues in aqueous electrolytes. Alternatively, manganese hexacyanomanganate was readily synthesized with high crystallinity and purity, resulting in a specific capacity of 57 mAh g −1 for its upper reaction. The lower reaction of this material (Mn II —N≡C—Mn II/I ) occurs at –0.612 V vs SHE, which is too low to allow efficient cycling in pH-neutral electrolytes without appreciable H 2 evolution. For these reasons, Mn II —N≡C—Mn III/II was selected as the anode to be used in full cells with the Cu II —N≡C—Fe III/II cathode. 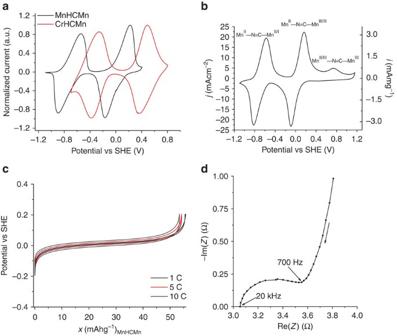Figure 3: Manganese hexacyanomanganate electrochemical characterization. (a) The cyclic voltammograms of manganese and chromium hexacyanomanganates in 10 M NaClO4pH=7 show two electrochemical processes in which the carbon-coordinated manganese reversibly changes its valence state between +1/+2 and +2/+3, respectively. (b) When cycled at higher potentials manganese hexacyanomanganate shows an additional, irreversible electrochemical process attributed to the oxidation of the N-coordinated Mn from +2 to +3. Galvanostatic cycling (c) at different C rates shows very low hysteresis resulting in high energy efficiencies, thanks to the low impedance of the system (d). Figure 3: Manganese hexacyanomanganate electrochemical characterization. ( a ) The cyclic voltammograms of manganese and chromium hexacyanomanganates in 10 M NaClO 4 pH=7 show two electrochemical processes in which the carbon-coordinated manganese reversibly changes its valence state between +1/+2 and +2/+3, respectively. ( b ) When cycled at higher potentials manganese hexacyanomanganate shows an additional, irreversible electrochemical process attributed to the oxidation of the N-coordinated Mn from +2 to +3. Galvanostatic cycling ( c ) at different C rates shows very low hysteresis resulting in high energy efficiencies, thanks to the low impedance of the system ( d ). Full size image The manganese hexacyanomanganate anode Mn II —N≡C—Mn III was synthesized by precipitation from aqueous precursors at room temperature (see methods section). The as-synthesized material has a composition of K 0.11 Mn[Mn(CN) 6 ] 0.83 · 0.17 ·3.64H 2 O ( =Mn(CN) 6 vacancy) as determined by CHN analysis and ICP-MS. X-ray diffraction of the fresh powders of both Cu II —N≡C—Fe III and Mn II —N≡C—Mn III revealed that they both have the FCC Prussian Blue crystal structure [27] . Their fully indexed diffraction spectra are shown in Fig. 2a,d . In both cases, the lattice parameter is consistent with those previously reported for these materials [39] . SEM showed that the morphology of the Prussian Blue analogues reported here varied with composition. The Mn II —N≡C—Mn III/II anode is composed of large, faceted particles 0.5–2 μm diameter ( Fig. 2b,c ), while the Cu II —N≡C—Fe III/II cathode is composed of polydisperse nanoparticles about 50 nm in size ( Fig. 2e,f ). The anode material precipitated more slowly during synthesis than the cathode material, resulting in the growth of fewer, but larger particles. As will be shown below, the high crystallinity and small particle size of OF materials aid rapid charge transport into each particle, allowing complete charge and discharge of these materials in short times. The OF materials were processed into electrodes using the standard slurry method widely practiced by the lithium-ion battery research community and manufacturers. These working electrodes were studied in aqueous flooded cells that also contained a Ag/AgCl/3.5M KCl reference electrode and an activated carbon counter electrode. Figure 3b shows the cyclic voltammogram of manganese hexacyanomanganate in 10 M NaClO 4 , pH=7 electrolyte. We postulate that both of the reactions observed for the hexacyanomanganate-based anodes are due to the electrochemical activity of the hexacyanomanganate groups and not the P-site nitrogen-coordinated manganese. For nearly every electrochemically active OF materials, it is the hexacyanometallate group, and not the nitrogen-coordinated P site metal cation, that is active. For example, the only electrochemical activity observed for chromium(III) hexacyanoferrate (Cr III —N≡C—Fe III/II ) is that of the hexacyanoferrate group, and, even at very low potentials, the chromium is not reduced [37] . During this study, we found that chromium in chromium(II) hexacyanoferrate (Cr II —N≡C—Fe III/II ) is also electrochemically inactive at low potentials. Among the numerous hexacyanoferrate-based cathodes, the exceptions to this rule are regular Prussian Blue (Fe III/II —N≡C—Fe III/II ) and hexacyanoferrates of vanadium ((V IV O) [2] + /V III —N≡C—Fe III/II ) [40] , titanium ((Ti IV O) [2] + /V III —N≡C—Fe III/II ) [41] and manganese (Mn III/II —N≡C—Fe III/II ) [37] . The materials containing vanadium and titanium are special cases, as the mechanism of their electrochemical activity is complicated by the formation of oxymetal cations. In the case of Mn III/II —N≡C—Fe III/II , the P-site manganese is electrochemically active only at high potentials near 1.0 V vs SHE [37] . In one recent study, Asakura et al . [42] found the manganese hexacyanomanganate anode to have two reaction potentials, one near 0.0 V vs SHE and the other near 0.7 V vs SHE, when the material was initially synthesized in a fully-reduced, low vacancy state containing only Mn 2+ (K 1.72 Mn[Mn(CN) 6 ] 0.93 · 0.07 ·0.65 H 2 O, green) . In this study, we also observed both of these two reactions, plus an additional peak at −0.7 V vs SHE ( Fig. 3b ). In our investigation the oxidation/reduction of manganese in the P-site was not reversible due to the high solubility and chemical instability of Mn III (Mn III —N≡C—Mn III ) in water-based electrolytes. Asakura et al . [42] observed a reversible phase change from cubic to monoclinic during cycling of the peak that they observed near 0.0 V vs SHE. However, we found that chemical reduction of the as-synthesized Mn II —N≡C—Mn III (light brown) to Mn II —N≡C—Mn II (Na 0.80 K 0.06 Mn[Mn(CN) 6 ] 0.83 · 0.17 ·2.17 H 2 O, light blue) using sodium dithionate Na 2 S 2 O 6 (E 0 =−0.66V) resulted only in a small change in lattice parameter and not in substantial changes to the FCC structure ( Fig. 4b ). 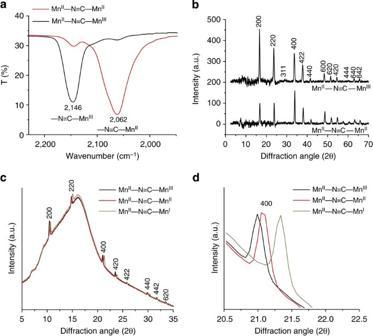Figure 4: Manganese hexacyanomanganate physical characterization. (a) Fourier transform infrared spectroscopy of oxidized MnII—N≡C—MnIIIand reduced MnII—N≡C—MnIIconfirm that the C-coordinated manganese is changing valence state. Thein situsynchrotron X-ray diffraction experiment (c,d) shows no change in crystal structure for MnII—N≡C—MnIII, MnII—N≡C—MnIIand MnII—N≡C—MnIexcept for a small peak shift corresponding to a decrease in lattice parameter during reduction. The broad background peak is due to the scattering by the water electrolyte (Supplementary Information). These results are confirmed by X-ray Powder Diffraction spectra (b) of oxidized MnII—N≡C—MnIIIand reduced MnII—N≡C—MnII. Figure 4: Manganese hexacyanomanganate physical characterization. ( a ) Fourier transform infrared spectroscopy of oxidized Mn II —N≡C—Mn III and reduced Mn II —N≡C—Mn II confirm that the C-coordinated manganese is changing valence state. The in situ synchrotron X-ray diffraction experiment ( c , d ) shows no change in crystal structure for Mn II —N≡C—Mn III , Mn II —N≡C—Mn II and Mn II —N≡C—Mn I except for a small peak shift corresponding to a decrease in lattice parameter during reduction. The broad background peak is due to the scattering by the water electrolyte ( Supplementary Information ). These results are confirmed by X-ray Powder Diffraction spectra ( b ) of oxidized Mn II —N≡C—Mn III and reduced Mn II —N≡C—Mn II . Full size image Physical characterization of MnHCMn at various oxidation states was performed in an effort to understand the mechanism of its electrochemical activity. The bonding in the Mn II —N≡C—Mn III structure was examined using Fourier Transform Infrared Spectroscopy (FTIR) ( Fig. 4a ). The infrared stretching frequencies of M-C bonds in the Prussian Blue structure are typically about 2,100 cm −1 . The stretching frequency of Mn III -C in freshly synthesized Mn II —N≡C—Mn III was found to be 2,146 cm −1 . After chemical reduction by Na 2 S 2 O 6 , the stretching frequency of Mn II -C in Mn II —N≡C—Mn II was found to be 2,062 cm −1 . Both of these values are in close agreement with those previously reported for a C-coordinated manganese, thus supporting our hypothesis that the electrochemical activity near 0 V is due to the hexacyanomanganate groups [39] . The X-ray photoelectron spectroscopy (XPS) ( Supplementary Fig. S3 ) and transmission electron microscopy electron energy loss spectroscopy (TEM EELS) ( Supplementary Fig. S5 ) spectra of the as-synthesized Mn II —N≡C—Mn III and the chemically reduced Mn II —N≡C—Mn II powders were also measured, but because of reasons described in the Supplementary Information it was not possible to ascribe the reduction to a specific manganese site. On the basis of these FTIR and electrochemical data, we therefore conclude that the redox behaviour of manganese hexacyanomanganate proceeds by the following mechanisms: The P-site manganese is electrochemically active around 0.7 V vs SHE (Equation 2). The hexacyanomanganate group is then reduced near 0 V vs SHE (Equation 3). In the first study to document the electrochemical activity of hexacyanomanganate-based Prussian Blue analogues, Scholz and Dostal proposed that the lowest reaction of these materials was due to the further reduction of hexacyanomanganate(II) to hexacyanomanganate(I). The exceedingly rare Mn(I) state is known to occur only in a few organometallic complexes, in the presence of very soft ligands like CO or CN. In fact, K 5 Mn(CN) 6 has been previously synthesized by chemical reduction of K 4 Mn(CN) 6 using aluminum as a reducing agent [43] , [44] , [45] . The mechanism for this reaction is shown in Equation 4: In situ synchrotron X-ray diffraction ( Fig. 4b,c and Supplementary Fig. S1 ) showed that during the reversible electrochemical processes (2) and (3), the material retains its face-centred cubic crystal structure and the lattice parameter decreases from 10.696 Å for the as-synthesized Mn II —N≡C—Mn III to 10.653 and 10.530 Å for Mn II —N≡C—Mn II and Mn II —N≡C—Mn I , respectively. We believe that this unusual behaviour corresponds to a decrease in the radius of [Mn III (CN) 6 ] 3− ions during their reduction to [Mn II (CN) 6 ] 4− and [Mn I (CN) 6 ] 5− , as previously demonstrated in the case of hexacyanoferrates [46] . Safety considerations Further physical characterization of the Cu II —N≡C—Fe III/II cathode and the Mn II —N≡C—Mn III/II anode was performed with thermogravimetric analysis mass spectroscopy (TGA-MS). Both materials were found to lose about 25% water ( Fig. 5 ). This accounts for the discrepancy between the observed specific capacities of Prussian Blue analogues in aqueous cells (~60 mAh g −1 ) and the theoretical capacities calculated from the anhydrous chemical formulae (~80 mAh g −1 ). In addition, both materials were found to be quite stable against HCN release. The Cu II —N≡C—Fe III cathode did not begin to release HCN until 200 °C, which is also the reported decomposition temperature for potassium ferricyanide. The Mn II —N≡C—Mn III anode did not begin to release HCN until 120 °C, a temperature higher than that at which aqueous batteries fail due to electrolyte evaporation. When reduced, both Cu II —N≡C—Fe II and Mn II —N≡C—Mn II show improved thermal stability. These TGA-MS results can be interpreted in terms of the strength of the N≡C—M bond: the N≡C—Fe bond is much stronger than the N≡C—Mn bond, and therefore more stable [45] . At the same time, a soft ligand like CN forms stronger bonds with softer ions, hence it loses stability when bonded to high oxidation state cations. In summary, thermal stability analysis using TGA-MS showed that these materials are safe for use in practical batteries for many stationary and portable applications. 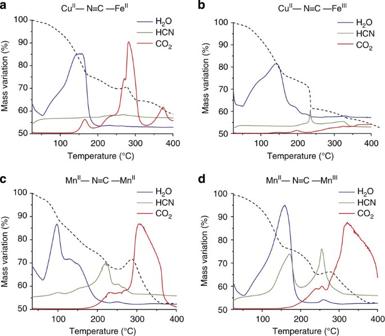Figure 5: Electrode materials thermal stability. Thermogravimetric analysis-mass spectrometry (TGA-MS) under inert (N2) atmosphere of (a) reduced (CuII—N≡C—FeII) and (b) oxidized (CuII—N≡C—FeIII) copper hexacyanoferrate shows that these materials is about 25 wt% of water and that HCN is not released from the structure for temperatures higher than 200 °C. Because of the lower stability of the Mn-C bond, (c) reduced (MnII—N≡C—MnII) and (d) oxidized (MnII—N≡C—MnIII) manganese hexacyanomanganate release HCN starting from 120 °C, temperature high enough for a water-based electrolyte. As general trend, the lower is the oxidation state, the higher is the stability of the material being CN a soft base it forms a stronger bond with soft metals, therefore with a lower oxidation state. Figure 5: Electrode materials thermal stability. Thermogravimetric analysis-mass spectrometry (TGA-MS) under inert (N 2 ) atmosphere of ( a ) reduced (Cu II —N≡C—Fe II ) and ( b ) oxidized (Cu II —N≡C—Fe III ) copper hexacyanoferrate shows that these materials is about 25 wt% of water and that HCN is not released from the structure for temperatures higher than 200 °C. Because of the lower stability of the Mn-C bond, ( c ) reduced (Mn II —N≡C—Mn II ) and ( d ) oxidized (Mn II —N≡C—Mn III ) manganese hexacyanomanganate release HCN starting from 120 °C, temperature high enough for a water-based electrolyte. As general trend, the lower is the oxidation state, the higher is the stability of the material being CN a soft base it forms a stronger bond with soft metals, therefore with a lower oxidation state. Full size image Dehydrated perchlorate salts do pose flammability hazards, but in aqueous solutions they are not hazardous. In particular, sodium perchlorate is highly hygroscopic, having one of the highest solubilities of any sodium salt in water. Replacement of perchlorate with an even more benign sodium salt will be a topic of future study. Full batteries containing a Cu II —N≡C—Fe III/II cathode, a Mn II —N≡C—Mn III/II anode and excess 10 M NaClO 4 electrolyte were characterized using galvanostatic cycling. In such cells, the cathode operates between 1.15 and 0.85 V vs SHE, while the anode operates between –0.2 V and 0.2 V ( Fig. 6a ). This results in a full cell that operates between 1.35 and 0.65 V, with an average discharge voltage of 0.95 V. Although this cell voltage is lower than those of commercial lithium-ion and lead acid cells, it is comparable to the nominal voltages of vanadium redox flow batteries. Because of the high ionic conductivity of the electrolyte and rapid reaction of the electrodes, very little voltage hysteresis occurs during fast charge and discharge, and little of the nominal voltage of the cell is lost even at a 6 min (10C) cycling rate ( Fig. 6b ). The low voltage hysteresis observed during rapid cycling, along with a high coulombic efficiency of over 99.9%, results in a very high round trip energy efficiency: 95.4% at a 10C rate and 84.2% even at a 50C rate ( Fig. 6c ). Finally, the very low full cell impedance ( Fig. 6d ) and low voltage hysteresis of this battery allow much of its low-rate capacity to be utilized at high rates. At a 10C rate, 92.9% of the maximum discharge capacity was retained above 0.65 V, while at a 50C rate, 73.3% was still available. 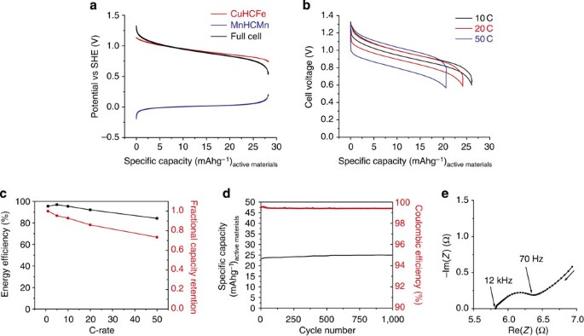Figure 6: Full cell electrochemical characterization. (a) Potential profiles of the copper hexacyanoferrate (CuII—N≡C—FeIII/II) positive electrode, the manganese hexacyanomanganate (MnII—N≡C—MnIII/II) negative electrode and the full cell voltage at a 1C rate. (b) The full cell voltage profiles at different C rates (10C, 20C, 50C). (c) Energy efficiency and fractional capacity retention as a function of C rate. (d) Cycling of the CuII—N≡C—FeIII/II- MnII—N≡C—MnIII/IIcell at a rate of 10C showed no capacity loss after 1,000 cycles and a coulombic efficiency of 99.8%. (e) The specific energy vs specific power plot shows intermediate performance between lithium ion batteries and ultracapacitors, ideally positioning this technology for short-term grid-scale energy storage, especially to handle transients. Figure 6: Full cell electrochemical characterization. ( a ) Potential profiles of the copper hexacyanoferrate (Cu II —N≡C—Fe III/II ) positive electrode, the manganese hexacyanomanganate (Mn II —N≡C—Mn III/II ) negative electrode and the full cell voltage at a 1C rate. ( b ) The full cell voltage profiles at different C rates (10C, 20C, 50C). ( c ) Energy efficiency and fractional capacity retention as a function of C rate. ( d ) Cycling of the Cu II —N≡C—Fe III/II - Mn II —N≡C—Mn III/II cell at a rate of 10C showed no capacity loss after 1,000 cycles and a coulombic efficiency of 99.8%. ( e ) The specific energy vs specific power plot shows intermediate performance between lithium ion batteries and ultracapacitors, ideally positioning this technology for short-term grid-scale energy storage, especially to handle transients. Full size image Extended cycling of full batteries containing a Cu II —N≡C—Fe III/II cathode and a Mn II —N≡C—Mn III/II anode was also performed. After 1,000 cycles at a 10C rate, there was no measurable capacity loss ( Fig. 6d ). The coulombic efficiency during extended cycling was 99.8%. In summary, this novel, symmetric open-framework electrode battery delivers a maximum specific energy of 27 Wh kg −1 at a 1C rate on a basis of the masses of the active materials. Furthermore, this battery has a specific energy of 15 Wh kg −1 , a specific power of 693 W kg −1 and an 84.2% energy efficiency when cycled at a 50C rate. These properties, together with the outstanding cycle life and low active materials cost, make this battery attractive for grid-related applications, including the smoothing of intermittent variations in power production associated with the integration of renewable energy on the grid. Copper hexacyanoferrate synthesis Preparation of nanoparticulate copper hexacyanoferrate was based on our recently reported synthesis procedures [7] . In brief, equal volumes of 40 mM Cu(NO 3 ) 2 (Alfa Aesar) and 20 mM K 3 Fe(CN) 6 (Sigma Aldrich) were combined by simultaneous, dropwise addition into water under vigorous stirring. An excess of Cu +2 is necessary for precipitation and particle growth. All of the Fe(CN) 6 is oxidized initially, but fully charged Cu II —N≡C—Fe III has a potential high enough to oxidize water. Thus, spontaneous partial reduction of Cu II —N≡C—Fe III occurs, resulting in a fractional initial charge state, typically about 80%. Five minutes after complete addition of the Cu II —N≡C—Fe III precursors, 0.1 M Na 2 S 2 O 3 was added until a desired molar ratio of Fe III (CN) 6 −3 to S 2 O 3 −2 was reached. The colour of Cu II —N≡C—Fe II changed from tan to purple upon addition of Na 2 S 2 O 3 , indicating a successful reduction. The CuHCF was filtered, washed with water and dried in vacuum at room temperature. Manganese hexacyanomanganate synthesis A similar preparation method was used for manganese (II) hexacyanomanganate (III). 0.5 g (15 mmol) of solid K 3 Mn(CN) 6 was added to a 50 ml solution of 0.1 M Mn(NO 3 ) 2 (50 mmol) using ultrapure distilled water, in a dark container, under vigorous stirring for 20 min. The resulting light brown precipitate was washed and centrifuged three times with 25 ml of water and then two more times with 25 ml of acetonitrile before being dried under vacuum at room temperature. The chemically-reduced manganese(II) hexacyanomanganate(II) was obtained by reduction of Mn II —N≡C—Mn III with a 0.1 M solution of sodium tetrathionate. Chromium hexacyanomanganate synthesis To synthesize chromium (II) hexacyanomanganate (III), 0.5 g of CrCl 2 was dissolved in 35 ml H 2 O. 0.5 g K 3 Mn(CN) 6 dissolved in 20 ml of 10 mM KCN solution and then added to the CrCl 2 solution and stirred for 3 h in a dark container. The excess CN − from the KCN helped to slow hydrolysis of the Cr 2+ . The resulting dark brown powder was centrifuged and washed three times in water, followed by a final wash in methanol, before being dried in vacuum at room temperature. Electrodes preparation Slurries containing Cu II —N≡C—Fe II or Mn II —N≡C—Mn III amorphous carbon (Super P Li), poly(vinylidene) difluoride (PVDF, Kynar HSV900) and graphite (Timcal KS6) in a ratio of 80:9:9:2 were prepared by grinding these materials by hand and then dispersing them in 1-methyl-2-pyrolidinone (NMP). Electrodes with mass loadings of about 10 mg cm −2 were prepared by spreading the slurry on a carbon cloth current collector (Fuel Cell Earth/Ballard Avcarb). The electrodes were dried in vacuum at 60 °C for 1 h. Electrochemical cell setup Flooded full cells containing a CuHCF cathode, an MnHCMn anode, 10 M sodium perchlorate electrolyte saturated with Mn(ClO 4 ) 2 at pH=6.4 and a Ag/AgCl 3.5 M reference electrode were prepared in a nitrogen-filled glove box. The presence of Mn(ClO 4 ) 2 in solution further decrease the solubility of MnHCMn in the electrolyte, thus resulting in improved cycle life performance. Moreover, the addition of Mn(ClO 4 ) 2 in the solution results in the precipitation of Mn(OH) 2 that buffer the pH at 6.4. The MnHCMn electrode is sensitive to oxidation, hence the cell must be kept oxygen-free to achieve efficient anode cycling at potentials below the SHE. How to cite this article: Pasta, M. et al . Full open-framework batteries for stationary energy storage. Nat. Commun. 5:3007 doi: 10.1038/ncomms4007 (2014).